Tailoring the graphene/silicon carbide interface for monolithic wafer-scale electronics Graphene is an outstanding electronic material, predicted to have a role in post-silicon electronics. However, owing to the absence of an electronic bandgap, graphene switching devices with high on/off ratio are still lacking. Here in the search for a comprehensive concept for wafer-scale graphene electronics, we present a monolithic transistor that uses the entire material system epitaxial graphene on silicon carbide (0001). This system consists of the graphene layer with its vanishing energy gap, the underlying semiconductor and their common interface. The graphene/semiconductor interfaces are tailor-made for ohmic as well as for Schottky contacts side-by-side on the same chip. We demonstrate normally on and normally off operation of a single transistor with on/off ratios exceeding 10 4 and no damping at megahertz frequencies. In its simplest realization, the fabrication process requires only one lithography step to build transistors, diodes, resistors and eventually integrated circuits without the need of metallic interconnects. Graphene has outstanding electronic properties [1] , [2] , [3] , namely excellent charge-carrier mobilities up to the order of 10 6 cm 2 Vs −1 (ref. 4 ), extremely high current stability in excess to 4-6 mA μm −1 (refs [5] , [6] 5,6), high-temperature stability and high thermal conductivity [7] . These properties make it appealing for applications in electronics. The most immediate applications employ its (semi-)metallic character, for example, as transparent conductive layer, for example, for displays and solar cells. Further, the rather weak switching properties in graphene transistors can be used for analogue amplification at high frequencies [8] . However, the use of graphene in replacement for a semiconductor fails because of the absence of an electronic bandgap [9] , [10] . Many efforts have been undertaken to establish a gap in graphene devices, with a bandgap induced by bilayer graphene [11] , [12] , [13] , [14] , [15] , spatial confinement [16] , [17] , [18] , localization [19] , [20] and chemical treatment [20] , [21] , resulting in rather small effects remote from technical requirements. It is an open question whether the excellent capabilities of graphene can be maintained after such a modification. We focus on epitaxial graphene on 6H silicon carbide (SiC) (0001), which provides excellent quality [22] and semiconductor technology compatible processing on the wafer scale [8] . Up to now in graphene experiments mainly semi-insulating SiC has been used to suppress all current paths through the substrate. SiC, as active component of the system, has been widely disregarded. It is a wide bandgap semiconductor for applications in high-voltage and high-power electronics [23] , [24] , [25] , [26] . Its material properties have been thoroughly investigated [27] , [28] , [29] and devices are commercially available. The material combination graphene on SiC thus combines two of the most robust materials for electronic applications we are aware of [5] , [30] , [31] and both materials are in intimate, epitaxially defined contact. In most cases, this contact leads to the formation of a Schottky barrier, with graphene as the metal and SiC as the semiconductor [32] , which allows basically no exchange of charge carriers. However, this interface can be tailored as an electronically transparent ohmic contact. We demonstrate a device concept based on a suitable combination of these interfaces. We present a simple fabrication strategy, which leads to normally-on and normally-off transistors. The measurements indicate that they are well suited as fast and efficient switches. In a further step, a complete logic is envisaged. 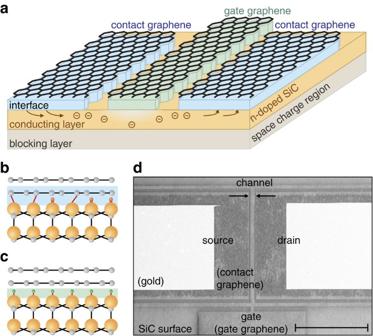Figure 1: Two different epitaxial graphene materials combined to a monolithic transistor. We consider the entire system epitaxial graphene employing its constituent graphene, SiC and their common interface. The wide bandgap semiconductor SiC forms the transistor channel. (a) Schematic of the device. Out of a single layer of graphene, two different interfaces are tailored side by side, resulting in ohmic contact graphene for source and drain (b), and Schottky-like gate graphene (c). The currents are guided in two layers from the graphene source through the semiconducting channel to the graphene drain. The channel conductance is modulated by the top-gate voltage. (d) An electron micrograph showing the device geometry. Contact graphene and gate graphene can be distinguished by different grey scales. Scale bar, 100 μm. Device concept and implementation Figure 1a shows the essential device concept of a single transistor, similar to a metal-semiconductor field-effect transistor: graphene forms the source, drain and gate electrode, and the SiC substrate is the semiconducting transistor channel. In this concept, we intend to guide the current in two layers: charge flows to the transistor in the graphene layer and the semiconducting layer provides the switch to carry the charge from source to drain, when the channel is open. Hence, we need a graphene layer with good charge carrier injection into SiC, which we call 'contact graphene'. It turns out that when growing graphene out of n-type SiC (by thermal decomposition [33] ), the resulting material combination n-type monolayer graphene (MLG) and n-type SiC is one of the few favourable solutions [34] for this problem. In MLG, as depicted in Fig. 1b , an electrically active graphene layer with a useful electron density n and mobility μ ( n= 10 13 cm −2 , μ e =900 cm 2 Vs −1 at room temperature) resides on a so-called buffer layer of carbon with R30 symmetry, which is electrically inactive. The outmost Si atoms of the SiC form partly covalent bonds to the buffer layer, partly they have dangling bonds under the buffer layer, which provide Fermi level pinning of the graphene electron system. We will demonstrate that this interface is a good choice for contact graphene. For the gate electrode, however, a good insulation is necessary. This 'gate graphene' can be implemented in many ways [35] , [36] . We opted for quasi-freestanding bilayer graphene (QFBLG, see Fig. 1c ) on the same n-type SiC, which is obtained from MLG material by hydrogen intercalation [37] . During this conversion (typically in H 2 atmosphere at 850 °C), the covalent bonds between SiC and graphene break up and the dangling bonds are saturated with hydrogen atoms. The buffer layer converts to an additional graphene layer. The result is a positively charged graphene bilayer with hole density p =10 13 cm −2 , μ h =2,000 cm 2 Vs −1 at room temperature. As QFBLG forms a Schottky contact with SiC, it serves well as gate graphene. Figure 1: Two different epitaxial graphene materials combined to a monolithic transistor. We consider the entire system epitaxial graphene employing its constituent graphene, SiC and their common interface. The wide bandgap semiconductor SiC forms the transistor channel. ( a ) Schematic of the device. Out of a single layer of graphene, two different interfaces are tailored side by side, resulting in ohmic contact graphene for source and drain ( b ), and Schottky-like gate graphene ( c ). The currents are guided in two layers from the graphene source through the semiconducting channel to the graphene drain. The channel conductance is modulated by the top-gate voltage. ( d ) An electron micrograph showing the device geometry. Contact graphene and gate graphene can be distinguished by different grey scales. Scale bar, 100 μm. Full size image An additional challenge is to combine both graphene species side-by-side on a single chip. We start with 6H-SiC (0001), entirely covered with contact graphene. To avoid a complete conversion of the graphene layer, we carry out the hydrogen intercalation process at a reduced temperature. As a consequence, no conversion to gate graphene takes place on the impenetrable graphene surface. However, at lithographically defined edges of the graphene sheet, or at voids, hydrogen can intercalate from the side and slowly converts contact graphene to gate graphene. We have found robust parameter sets for penetration depths d p from 350 nm to 1.5 μm, with no indication for a lower limitation. For the given structure size, T =540 °C with d p =500 nm was adequate. This kinetically controlled process can be used to partially convert small gate structures into gate graphene, whereas the larger source and drain electrodes remain contact graphene, except at their edges. When large area gate graphene is required, a perforation previous to hydrogen treatment is used, in particular for the gate electrode's contact pad. Hence, using a single chip of as-grown graphene, after only one lithography step, we can define two interface functionalities by geometry: contact graphene and gate graphene side-by-side. For our actual research, we used a second lithography step to reduce partially converted areas at the edges of the contact graphene, to ensure well-defined conditions. The two different materials can be distinguished in standard electron microscope images as different grey scales ( Fig. 1d ). On the stepped off-axis substrate required for epitaxial growth of the pn layers (see below), additionally an undesired conversion to gate graphene occurs along the substrate steps that causes the stripes in the contact graphene areas. Further, we have to take care for a geometric confinement of the channel in the semiconductor. A vertical confinement is predefined by an epitaxially grown layered pn junction [38] that leaves the top surface of the wafer as low doped conducting n-type layer of 2.9 μm depth (out of which graphene is grown). The space charge region of the pn junction suppresses any charge carrier density below this conducting layer. By applying a parametric backgate voltage, the thickness of the space charge region and, complementary, the thickness of the conducting layer can be varied in operandi . It should be stressed that the backgate is a convenient control parameter for our test system, but is not required for the device operation, when doping and thickness of the n-type epilayer are well balanced. Laterally, the channel is confined such that the gate separates the source and drain contact. This is necessary for low off-current level and to avoid crosstalk between two transistors. Properties of contact graphene and gate graphene First, we verified the electrical contact properties of the two different graphene/SiC interfaces. 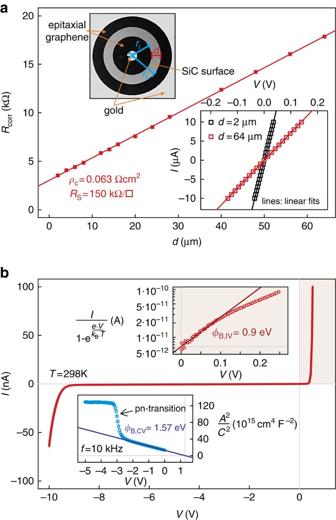Figure 2: Characterization of graphene/silicon carbide contacts. (a) We have characterized the ohmic contacts of MLG on SiC. The left inset shows the geometry of the CTLM pattern. The grey ring corresponds to the SiC channel with parametrically varied lengthd. The inner and outer parts are used as contacts. The right inset corroborates the linearity of theI–Vcharacteristics (ohmic contacts), despite a very low doping of the semiconductor. The slopeRcorr(corrected for cylindric geometry39) of the correspondingI–Vcurves is plotted againstdin the main figure. From the linearRcorr(d) dependence contact and sheet resistance,ρCandRS, respectively, are derived. (b)I–Vcharacteristics of a QFBLG/SiC junction with ohmic counter electrode. The rectifying Schottky behaviour justifies the use as gate graphene. A Schottky barrier heightB,IV=0.9 eV is extracted from the forward characteristics (shaded area, same data shown in upper inset).B,CV=1.57 eV is extracted fromC–Vdata (lower inset) on the same device. Figure 2a displays room temperature resistance measurements taken on circular transfer length method (CTLM) structures fabricated of MLG (left inset) as a function of electrode spacing d . A geometry correction has properly been carried out, following the procedure of ref. 39 . Each data point corresponds to the slope of a linear I – V , two examples of which are shown in the right inset. No deviation from ohmic I – V s was found, even at lowest voltages. From the distance dependence (which is again perfectly linear), we can derive both the contact resistance of ρ C =0.063 Ωcm 2 and the sheet resistance R S ~150 kΩ/ of the n-type SiC layer, the latter in accordance with Hall measurements in a different sample without graphene ( μ SiC =370 cm 2 Vs −1 , n =1×10 15 cm −3 ). The remarkable feature of the graphene/SiC contact is its perfectly ohmic behaviour, despite the very low doping concentration of the SiC epilayer, which is absent for metallic contacts (in particular, annealed nickel contacts) on the very same material. The extracted value ρ C is on the first sight substantially higher than for state-of-the-art metal ohmic contacts to highly doped SiC [40] . However, by further CTLM measurements on highly nitrogen (N)-doped 6H SiC material (nitrogen concentration [N]=10 19 cm −3 ), we could verify that additional contact doping can improve ρ C by orders of magnitude: contact resistances of ρ C =6 μΩcm 2 were reached, which are well competitive with state-of-the-art ohmic contacts on SiC [41] (we currently run an extensive study on this item). There is an analogy to state-of-the-art metal ohmic contacts to SiC, where carbon is considered as an important mediator for transparent interfaces [42] . We conclude that MLG is ideally suited as contact graphene. Figure 2: Characterization of graphene/silicon carbide contacts. ( a ) We have characterized the ohmic contacts of MLG on SiC. The left inset shows the geometry of the CTLM pattern. The grey ring corresponds to the SiC channel with parametrically varied length d . The inner and outer parts are used as contacts. The right inset corroborates the linearity of the I – V characteristics (ohmic contacts), despite a very low doping of the semiconductor. The slope R corr (corrected for cylindric geometry [39] ) of the corresponding I – V curves is plotted against d in the main figure. From the linear R corr ( d ) dependence contact and sheet resistance, ρ C and R S , respectively, are derived. ( b ) I – V characteristics of a QFBLG/SiC junction with ohmic counter electrode. The rectifying Schottky behaviour justifies the use as gate graphene. A Schottky barrier height B,IV =0.9 eV is extracted from the forward characteristics (shaded area, same data shown in upper inset). B,CV =1.57 eV is extracted from C – V data (lower inset) on the same device. Full size image Similarly, we carried out C – V and I–V measurements on QFBLG contacts on the same SiC material equipped with ohmic nickel counter electrodes ( Fig. 2b ), resulting in a rectifying behaviour. We could derive a lower limit of the injection barrier B,IV =0.9 eV from the I – V measurements (upper inset) and an upper limit B,CV =1.1 eV ... 1.6 eV from C – V measurements (lower inset), using a standard evaluation [43] . These values are comparable to those of metals in contact with SiC [44] . Hence, QFBLG forms the desired Schottky contact to n-type SiC, which justifies its use as gate graphene. However, the spread of resulting Schottky barrier heights obtained from these two methods and the sample-to-sample fluctuations indicate that this barrier strongly depends on surface quality and may be improved by better process control. Transistor operation In a next step, we defined a transistor ( Fig. 1 ) with contact graphene source and drain electrodes and a top-gate electrode made out of gate graphene. We investigated the response of the source-drain current I D on variation of the following parameters: source-drain voltage, V SD ; top-gate voltage, V TG ; back-gate voltage, V BG ; and temperature, T . 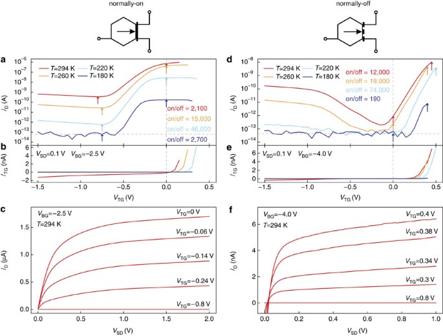Figure 3: Electrical characterization of a monolithic epitaxial graphene transistor. Transfer characteristics (a) and gate leakage currents (b) for various temperatures, and output characteristics (c) at room temperature in the normally-on operation mode. On/off ratios were determined between the current at top-gate voltageVTG=0 V and the minimum drain currentIDvalue (indicated by arrows). (d–f) Corresponding plots for normally-off operation mode. The current contributionIDincreasing towards more negativeVTGcan be identified as leakage currentITG, which depends on interface quality. In both modes, the largest on/off contrast is achieved atT=220 K. We present the data in two specific regimes defined by V BG : normally-on and normally-off operation indicated by the switch state at V TG =0 V. Figure 3a displays the transfer characteristic in the normally-on regime, which was achieved at V BG =−2.5 V. In this state, at V TG =0 V, the channel is open and the current I D between the two ohmic contacts is almost at its maximum value. When applying a negative V TG , the channel becomes depleted by the increasing space charge region of the Schottky contact, which reduces I D . At room temperature, this suppression leads to an on/off ratio of 2,100, with a minimum value of I D =0.36 nA at V TG =−0.8 V. This minimum value and the upturn at even lower V TG is governed by the leakage current I TG of the Schottky contact ( Fig. 3b ) owing to the rather small effective barrier B of this device. Consequently, the leakage current is strongly reduced towards lower temperatures. At T =220K, the minimal current I D is reduced to 0.6 pA leading to a very high on/off ratio of 46,000. The comparison of the transfer characteristics for different T is shown in Fig. 3a . With reduced T also the on-current is reduced because of charge carrier freeze-out in the SiC channel region [45] . Below 220K, this effect results in a reduction of the on/off contrast. This indicates that all curves are dominated by semiconductor material properties, which can be engineered by variation of the doping according to the requirements, and by the surface quality. Figure 3c displays the corresponding output characteristics at room temperature. We find a linear rise at low V SD and a quasi-saturated behaviour at higher values. The transistor withstands V SD =5 V without any irreversible change. Figure 3: Electrical characterization of a monolithic epitaxial graphene transistor. Transfer characteristics ( a ) and gate leakage currents ( b ) for various temperatures, and output characteristics ( c ) at room temperature in the normally-on operation mode. On/off ratios were determined between the current at top-gate voltage V TG =0 V and the minimum drain current I D value (indicated by arrows). ( d – f ) Corresponding plots for normally-off operation mode. The current contribution I D increasing towards more negative V TG can be identified as leakage current I TG , which depends on interface quality. In both modes, the largest on/off contrast is achieved at T =220 K. Full size image We now turn to the normally-off operation achieved at V BG =−4 V ( Fig. 3d–f ). Here at V TG =0 V, the channel is already switched off, because the space-charge regions of the unbiased graphene top-gate and of the pn junction back-gate meet. By applying a positive V TG , we reopen the channel for the source-drain current I D , thereby increasing I D by a factor of 12,000 at room temperature. This maximum is limited by the measurement compliance I TG < 10 nA: the disadvantage of this mode is, that the required positive V TG drives the Schottky gate in forward direction, as can be seen in the leakage current I TG in Fig. 3e . Again at negative V TG , I TG determines I D . Similar to the above reasoning, we try to reduce the influence of leakage by reducing T . The best on/off ratio with a value of 74,000 is again achieved at 220 K. The overall current levels I D are substantially smaller ( Fig. 3f ) compared with the normally on operation. For all characteristics, hysteresis was essentially absent. Switching speed As the device is a unipolar field-effect transistor, it is expected to switch fast [46] . Although our design did not target high-frequency operation (for example, we used large contact pads, conductive substrate), we measured the AC response I D ( f ) when a sinusoidal voltage V TG ( f ) was applied to the top-gate. No significant damping/phase shift and no signal distortion was observed up to 1 MHz. This observation corresponds well with textbook predictions for the cutoff frequency of a metal-semiconductor field-effect transistor [43] (at which the AC gate current I TG is equal to the drain current I D ): . Here g is the transconductance, which is extracted from the transfer characteristics of our device at room temperature, and C TG , the capacitance of the top-gate. In our proof-of-concept layout, the area that contributes to C TG is unnecessarily large as it includes the bond pad of the gate structure. As the simplest example for a design improvement, we could use semi-insulating SiC for the peripheral regions of the transistor (for example, by vanadium implantation). This should reduce C TG and consequently f T is supposed to increase by a factor of ~30. The route for further speed improvements is obvious: optimization and shrinkage of the geometry, reduction of source, drain resistances, and so on. In summary, we present an integrated scheme for a transistor with high on/off ratios using epitaxial graphene on 6H-SiC (0001). It is monolithic in the sense that it includes and relies on the entire system graphene, SiC and its interfaces, and furthermore, that devices can be carved out of a single epitaxial graphene/SiC chip. With appropriate adaptations, they can be fabricated side-by-side with present epitaxial graphene high-frequency architectures [8] (for which it provides the missing switch), and also with existing SiC high-power devices [23] , with low fabrication effort. We have reached on/off ratios up to 74,000 (or even more than 600,000 when comparing minimum and maximum current I D at U TG =−0.2 V and 0.6 V, respectively, for U BG =−3.5 V, U SD =1 V and T =220 K). We consider this device as a proof of concept. The presented device performance is not fundamentally limited and may be tailored according to specific requirements. In particular, the contact resistances can be improved by four orders of magnitude by contact implantation. Different intercalation conditions, variation of off-angle of the substrate, design optimisation, and so on, are expected to lead to uniform and therefore higher effective Schottky barriers. This will allow for higher currents, higher operation speed and higher operation temperatures. The concept's particular strength, however, lies in the following property: within the same processing steps, many epitaxial graphene transistors can be connected by graphene strip lines (the interface from contact graphene to gate graphene is electrically transparent [47] , [48] ) along with graphene resistors and graphene/SiC Schottky diodes ( Fig. 2b ), and therefore complex circuits can be built up. As a special feature of graphene in contrast to semiconductors, we anticipate that even a complete logic is feasible. Substrate and graphene growth A layered 6H-SiC pn junction with a 3-μm thick highly p-doped (2×10 18 cm −3 of aluminium) layer underneath a 2.9-μm thick slightly n-doped (1×10 15 cm −3 of nitrogen) layer was grown by means of chemical vapour deposition on top of a n-type 6H-SiC wafer 3.5° off the (0001) direction. After a hydrogen etch step (consuming 400 nm of SiC), graphene is grown by thermal decomposition of the SiC substrate at 1,650 °C under argon flux near room pressure [33] . Device fabrication Mesa structures are formed by reactive ion etching, using a lithographically defined mask of gold and nickel to separate the individual transistors and to give access to the p-doped layer. Mask residues were removed with aqueous KI:I 2 solution. To partly transform MLG to QFBLG, the samples were annealed in a rapid thermal annealing furnace at 540 °C and 880 mbar with a constant flux of 1 slm of purified hydrogen for 90 min. The conditions are chosen such that the hydrogen only intercalates through a regular pattern of small holes ( ~200 nm, distance 0.5 μm) prepared in the graphene layer, where conversion is desired. Subsequently, the devices are patterned by electron beam lithography and oxygen plasma etching. Titanium/gold contacts to the MLG and nickel contacts to the QFBLG regions are deposited by electron-beam evaporation and sputtering, respectively. The p-doped substrate layer is contacted via a large area nickel contact. Characterization The transistor characteristics were investigated in a continuous-flow cryostat with the sample in helium at 10 mbar using a Keithley 6430 source measurement unit with remote amplifier. Characterization of the contact properties was done in a Lakeshore probe station in vacuum using a 4-probe set-up using an Agilent E5270B measurement frame with 4 E5287A high-resolution source measurement modules and an Agilent E4980A LCR meter. How to cite this article: Hertel, S. et al . Tailoring the graphene/silicon carbide interface for monolithic wafer-scale electronics. Nat. Commun. 3:957 doi: 10.1038/ncomms1955 (2012).